Deranged fatty acid composition causes pulmonary fibrosis inElovl6-deficient mice Despite the established role of alveolar type II epithelial cells for the maintenance of pulmonary function, little is known about the deregulation of lipid composition in the pathogenesis of pulmonary fibrosis. The elongation of long-chain fatty acids family member 6 (Elovl6) is a rate-limiting enzyme catalysing the elongation of saturated and monounsaturated fatty acids. Here we show that Elovl6 expression is significantly downregulated after an intratracheal instillation of bleomycin (BLM) and in human lung with idiopathic pulmonary fibrosis. Elovl6 -deficient ( Elovl6 −/− ) mice treated with BLM exhibit severe fibroproliferative response and derangement of fatty acid profile compared with wild-type mice. Furthermore, Elovl6 knockdown induces a change in fatty acid composition similar to that in Elovl6 −/− mice, resulting in induction of apoptosis, TGF-β1 expression and reactive oxygen species generation. Our findings demonstrate a previously unappreciated role for Elovl6 in the regulation of lung homeostasis, and in pathogenesis and exacerbation of BLM-induced pulmonary fibrosis. Idiopathic pulmonary fibrosis (IPF) is a chronic interstitial lung disease characterized by fibroblast proliferation and excessive extracellular matrix deposition, resulting in severe respiratory insufficiency [1] , [2] . Increasing numbers of studies for the pathogenetic mechanism of IPF demonstrate notable roles of alveolar epithelial cell injury, which is triggered by various stimuli including oxidative stress and endoplasmic reticulum stress, and implies that accumulation of exceeding wound repair leads to a development of fibrosis [3] . The role of alveolar epithelial cell apoptosis during fibrosis has been extensively studied. For example, Plataki et al . [4] showed that the apoptosis promoting factors, p53, p21, Bax and caspase 3 were upregulated in bronchial and alveolar epithelial cells in lung specimens taken by biopsy in IPF patients, and TUNEL (terminal deoxynucleotide transferase-mediated deoxyuridine triphosphate-biotin nick end-labelling) was positive in alveolar epithelial cells of all IPF patients. Likewise, Kuwano et al . [5] demonstrated that caspase inhibitor protected progression of fibrosis in the rodent model. Moreover, alveolar epithelial cells produce transforming growth factor (TGF)-β1, which has a crucial role in lung fibrinogenesis [6] , [7] , [8] , [9] . Furthermore, the role of reactive oxygen species (ROS) and apoptosis in alveolar epithelial cells has been well appreciated as an initiation step of pulmonary fibrosis. However, the upstream mechanisms of ROS production and apoptosis in pulmonary fibrosis are still unclear. Therefore, the research to determine the molecular mechanisms underlying apoptosis and TGF-β production in alveolar epithelial cells may provide novel potential therapeutic targets for the treatment of IPF. The integrity of alveolar type II epithelial cells is indispensable for the maintenance of pulmonary function, partly because these cells synthesize pulmonary surfactant that is critical for lung compliance by facilitating the reduction of alveolar surface tension. Approximately 90% of surfactant consists of saturated phospholipids, of which phosphatidylcholine is by far the most abundant component with some triacylglycerols and cholesterol, and 10% of lung-specific surfactant proteins (SPs), SP-A, SP-B, SP-C and SP-D [10] . Surfactant deficiency or disruption of production of SPs results in alveolar damage [11] , [12] . A variety of mutations in the SP-C gene have been identified in patients with pulmonary fibrosis [13] , [14] . However, there is no evidence to date indicating that dysregulation of lipids components in alveolar type II epithelial cells predisposes the lung to injury and subsequent fibrotic response. Central to the lipid biosynthesis are the elongation and desaturation of fatty acids (FAs), which regulate the length and degree of unsaturation of FAs and thereby determine their function and metabolic fates. The elongation of long-chain FAs family member 6 (Elovl6) is a rate-limiting enzyme catalysing the elongation reaction of palmitate (C16:0) to stearate (C18:0), and stearate is converted to oleic acid (OA; C18:1n-9) by stearoyl CoA desaturase (SCD). Palmitate is converted to palmitoleic acid (C16:1n-7) by SCD, and palmitoleic acid is elongated to vaccenic acid (C18:1n-7) by Elovl6 or Elovl5 (refs 15 , 16 , 17 ). Matsuzaka et al . [15] demonstrated that Elovl6- deficient ( Elovl6 −/− ) mice are resistant to diet-induced insulin resistance, despite their hepatosteatosis and obesity being similar to that of the wild-type (WT) mice. Such a favourable metabolic response to high-fat diet in Elovl6 −/− mice may be largely due to increased ratio of palmitoleic acid to palmitic acid (PA) in the liver. More recent study has shown that atherogenic high-fat-diet-induced hepatic inflammation, oxidative damage and fibrosis in the liver were attenuated in Elovl6 −/− mice, despite comparable hepatosteatosis in Elovl6 −/− and WT mice [18] . These data suggest that alteration of FA components in Elovl6 −/− mice contribute to insulin sensitivity independently of obesity, cellular energy balance and stress. However, the effects of the change in FA composition in alveolar type II epithelial cells on their own homeostasis have not been investigated. In this study, we examine the effects of Elovl6 deficiency on the fibrotic response after bleomycin (BLM)-induced lung injury in vivo , and on apoptosis, TGF-β production and ROS production in alveolar type II epithelial cells in vitro . Our data using Elovl6 −/− mice provide a new role for Elovl6 by showing that Elovl6 deficiency promotes BLM-induced lung injury and makes alveolar type II epithelial cells more susceptible to oxidative stress. BLM treatment decreases Elovl6 expression in the lung To determine the expression of Elovl6 in the lung, we first carried out immunohistochemistry on lung tissue from untreated C57BL/6 (WT) control mice using anti-Elovl6 antibody and anti-SP-C antibody as an alveolar type II epithelial cell marker. As expected, control tissue show that SP-C is exclusively present in alveolar type II epithelial cells. Elovl6 staining appears to be similar to SP-C staining, suggesting that Elovl6 is expressed in alveolar type II epithelial cells ( Fig. 1a ). Next, we examined whether Elovl6 expression was affected during fibrotic change induced by intratracheal BLM instillation (1 mg kg −1 ). Histologic analysis at 21 days after BLM instillation demonstrated increased fibrosis, especially in peribronchial locations ( Fig. 1a ). Interestingly, Elovl6 staining was markedly reduced in epithelial cells, while SP-C staining was moderately reduced. We also measured the Elovl6 and SP-C mRNA expression in the lung from BLM-treated WT mice by quantitative reverse transcriptase–PCR (qRT–PCR). Elovl6 and SP-C mRNA levels were decreased by 42% and 20%, respectively, in the lung from BLM-treated mice compared with saline-treated control mice ( Fig. 1b,c ). Consistent with the results of qRT–PCR, elongase activity was decreased in lung of BLM-treated mice compared with that in WT lung ( Fig. 1d ). These data suggest that Elovl6 expression was preferentially downregulated in the alveolar type II epithelial cells in response to BLM. 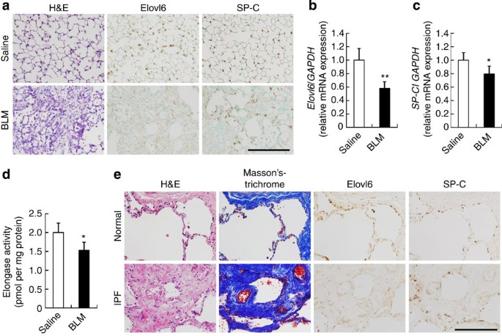Figure 1: Localization and expression of Elovl6 in BLM-treated mouse lung and in human lung with IPF. (a) Immunohistochemical staining with antibodies against Elovl6 and SP-C in lung sections from C57BL/6 mouse. H&E, haematoxylin and eosin. Expression of Elovl6 was colocalized with SP-C in alveolar epithelial cells in control mouse treated with saline (upper panels), and decreased in mouse treated with BLM 1 mg kg−1(lower panels) for 21 days. Scale bar, 200 μm. (b,c) qRT–PCR also showed lower expression ofElovl6andSP-CmRNA in mouse lung treated with BLM than control mice treated with saline.N=6 per group.GAPDHwas measured as an internal control. mRNA of the saline-treated group was normalized to a value of 1, and the mRNA level in the BLM-treated group is shown relative to the control level. Values are reported as the means±s.d. of three experiments. *P<0.05, **P<0.01 versus control, Mann–WhitneyU-test. (d) The Elovl6 enzymatic activity in lung microsomal fractions was significantly decreased in mice treated with BLM compared with mice treated with saline. Specific activity was expressed as pmol of radioactive [2-14C] malonyl-CoA incorporated into hydrophobic long-chain FA fractions by 1 mg of microsomal protein.N=4 per group. Values are reported as the means±s.d. of three experiments. *P<0.05 versus control, Student’st-test. (e) Immunohistochemical staining for Elovl6 and SP-C in lung specimen. Expression of Elovl6 was colocalized with SP-C in alveolar epithelial cells in normal lung area from lung cancer patient (upper panels), and decreased in fibrotic area from IPF patient (lower panels). Masson’s trichrome staining confirmed pulmonary fibrosis in IPF patient. Scale bar, 200 μm. Figure 1: Localization and expression of Elovl6 in BLM-treated mouse lung and in human lung with IPF. ( a ) Immunohistochemical staining with antibodies against Elovl6 and SP-C in lung sections from C57BL/6 mouse. H&E, haematoxylin and eosin. Expression of Elovl6 was colocalized with SP-C in alveolar epithelial cells in control mouse treated with saline (upper panels), and decreased in mouse treated with BLM 1 mg kg −1 (lower panels) for 21 days. Scale bar, 200 μm. ( b , c ) qRT–PCR also showed lower expression of Elovl6 and SP-C mRNA in mouse lung treated with BLM than control mice treated with saline. N =6 per group. GAPDH was measured as an internal control. mRNA of the saline-treated group was normalized to a value of 1, and the mRNA level in the BLM-treated group is shown relative to the control level. Values are reported as the means±s.d. of three experiments. * P <0.05, ** P <0.01 versus control, Mann–Whitney U -test. ( d ) The Elovl6 enzymatic activity in lung microsomal fractions was significantly decreased in mice treated with BLM compared with mice treated with saline. Specific activity was expressed as pmol of radioactive [2- 14 C] malonyl-CoA incorporated into hydrophobic long-chain FA fractions by 1 mg of microsomal protein. N =4 per group. Values are reported as the means±s.d. of three experiments. * P <0.05 versus control, Student’s t -test. ( e ) Immunohistochemical staining for Elovl6 and SP-C in lung specimen. Expression of Elovl6 was colocalized with SP-C in alveolar epithelial cells in normal lung area from lung cancer patient (upper panels), and decreased in fibrotic area from IPF patient (lower panels). Masson’s trichrome staining confirmed pulmonary fibrosis in IPF patient. Scale bar, 200 μm. Full size image Elovl6 expression is downregulated in the lung of patients with IPF To address the Elovl6 expression in the lung of IPF patients, we examined Elovl6 expression using immunohistochemistry on lung tissues from IPF patients and lung cancer patient. Immunoreactivity for Elovl6 localized to alveolar type II epithelial cell indicated by SP-C immunoreactivity in normal lung area of cancer patient. In the lung affected by IPF, Elovl6 expression was markedly decreased compared with SP-C expression ( Fig. 1e ). Elovl6 −/− knockout exacerbates pulmonary fibrosis by BLM To investigate the role of Elovl6 in fibrotic response in the lung, we compared the histopathology between Elovl6 −/− and WT mice with or without intratracheal instillation of BLM (1 mg kg −1 ) for 21 days. Haematoxylin and eosin and Masson’s trichrome staining revealed a modest but significant increase in fibrosis area in Elovl6 −/− mice compared with WT mice. As expected, intratracheal instillation of BLM induced prominent accumulation of collagen and extracellular matrix, thickened interalveolar septa and obstruction of alveolar space in WT mice at 21 days, and notably, such a response was markedly exaggerated in Elovl6 −/− mice ( Fig. 2a,b ). In addition, semiquantitative assessment using Ashcroft score demonstrated that BLM-induced pulmonary fibrosis was more extensive in the Elovl6 −/− lung than in WT lung ( Fig. 2c ). These histopathological changes were associated with increased mortality at 21 days after BLM instillation in Elovl6 −/− mice (6 of 28 mice in Elovl6 −/− mice versus 1 of 24 in WT mice). Elovl6 −/− mice weigh less than WT mice both before and 21 days after BLM administration (WT mice: before BLM, 25.2±1.0 and after BLM 26.3±1.4; Elovl6 −/− mice: before BLM, 22.0±1.5 and after BLM, 21.4±1.8; means±s.d.). Evaluation of collagen synthesis by sircol assay revealed that soluble collagen synthesis was significantly increased in Elovl6 −/− mice than in WT mice in response to BLM instillation ( Fig. 2d ). Consistent with these results, the procollagen type I and type III mRNA levels were robustly increased after BLM instillation in both WT and Elovl6 −/− lungs, and difference between these mice lungs did not reach statistical significance. Of note, smooth muscle α-actin gene expression was modestly but significantly elevated in Elovl6 −/− lung compared with WT lung at baseline and after BLM instillation, implying that lack of the Elovl6 gene per se promotes lung fibrosis ( Fig. 2e ). Taken together, these results suggest that deletion of the Elovl6 gene by itself induces a fibrotic change in the absence of BLM, and causes the life-threatening pulmonary fibrosis in response to BLM challenge in mice. 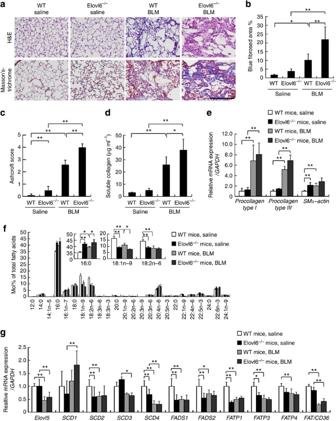Figure 2: Severity of pulmonary fibrosis rises inElovl6−/−mice exposed to BLM. (a–c) Masson’s trichrome staining (a) and semiquantitative analysis of fibrotic area (b), and Ashcroft score (c) in the lung. The area of pulmonary fibrosis and Ashcroft score were significantly increased inElovl6−/−mice treated with BLM in comparison with WT mice treated with BLM. Scale bar, 20 μm.N=6–8 per group. (d) Sircol assay showed that BLM induced soluble collagen synthesis in WT mice, and much higher inElovl6−/−mice than in WT mice.N=6 per group. (e) qRT–PCR analysis showed thatprocollagen type Iandtype IIImRNA expressions were markedly increased after BLM administration in WT orElovl6−/−mice. On the other hand,SMα–actinmRNA expression was significantly increased in saline-treatedElovl6−/−mice than in WT mice.N=4–5 per group. (f) FA composition of neutral lipid extract from the lung tissue. The relative amounts of PA (C16:0) was increased; in contrast, OA (C18:1n-9) or LA (C18:2n-6) were decreased inElovl6−/−mice compared with WT mice. The upper right diagrams were magnified figures of PA (C16:0), OA (C18:1n-9) and LA (C18:2n-6). Similar toElovl6−/−mice, the ratio of PA was increased. In contrast, OA and LA were decreased in WT mice treated with BLM. These changes of FA composition were more apparent inElovl6−/−mice treated with BLM.N=4 per group. (g) qRT–PCR of various mRNA levels involved with FA metabolism in WT andElovl6−/−mice lungs treated with saline or BLM.N=4–5 per group.GAPDHwas measured as an internal control. mRNA of the saline-treated group was normalized to a value of 1, and the mRNA levels in theElovl6−/−mice and BLM-treated group are shown relative to the control level. Inb–g, all values are represented as the means±s.d. of three experiments. *P<0.05, **P<0.01 versus WT/Elovl6−/−treated with saline or BLM (b–d,f), or WT/Elovl6−/−treated with saline (e,g), measured by Steel–Dwass (b,c,f) or Tukey–Kramer test (d,e,g). Figure 2: Severity of pulmonary fibrosis rises in Elovl6 −/− mice exposed to BLM. ( a – c ) Masson’s trichrome staining ( a ) and semiquantitative analysis of fibrotic area ( b ), and Ashcroft score ( c ) in the lung. The area of pulmonary fibrosis and Ashcroft score were significantly increased in Elovl6 −/− mice treated with BLM in comparison with WT mice treated with BLM. Scale bar, 20 μm. N =6–8 per group. ( d ) Sircol assay showed that BLM induced soluble collagen synthesis in WT mice, and much higher in Elovl6 −/− mice than in WT mice. N =6 per group. ( e ) qRT–PCR analysis showed that procollagen type I and type III mRNA expressions were markedly increased after BLM administration in WT or Elovl6 −/− mice. On the other hand, SMα–actin mRNA expression was significantly increased in saline-treated Elovl6 −/− mice than in WT mice. N =4–5 per group. ( f ) FA composition of neutral lipid extract from the lung tissue. The relative amounts of PA (C16:0) was increased; in contrast, OA (C18:1n-9) or LA (C18:2n-6) were decreased in Elovl6 −/− mice compared with WT mice. The upper right diagrams were magnified figures of PA (C16:0), OA (C18:1n-9) and LA (C18:2n-6). Similar to Elovl6 −/− mice, the ratio of PA was increased. In contrast, OA and LA were decreased in WT mice treated with BLM. These changes of FA composition were more apparent in Elovl6 −/− mice treated with BLM. N =4 per group. ( g ) qRT–PCR of various mRNA levels involved with FA metabolism in WT and Elovl6 −/− mice lungs treated with saline or BLM. N =4–5 per group. GAPDH was measured as an internal control. mRNA of the saline-treated group was normalized to a value of 1, and the mRNA levels in the Elovl6 −/− mice and BLM-treated group are shown relative to the control level. In b – g , all values are represented as the means±s.d. of three experiments. * P <0.05, ** P <0.01 versus WT/ Elovl6 −/− treated with saline or BLM ( b – d , f ), or WT/ Elovl6 −/− treated with saline ( e , g ), measured by Steel–Dwass ( b , c , f ) or Tukey–Kramer test ( d , e , g ). Full size image Elovl6 deficiency alters FA composition in vivo To explore the mechanisms by which Elovl6 deficiency aggravates pulmonary fibrosis with and without BLM instillation, we aimed to determine whether Elovl6 deficiency leads to alteration of FA composition in the lung. To this end, we extracted total lipids from the lung of WT or Elovl6 −/− mice and measured FA composition. As shown in Fig. 2f , relative amounts of C16-saturated FA, PA (C16:0), was increased, whereas C18 monounsaturated FA OA (C18:1n–9) was decreased. These results were consistent with the changes in hepatic FA composition in the chow-fed Elovl6 −/− mice as reported by Matsuzaka et al . [15] Interestingly, FA composition in the lung from untreated Elovl6 −/− mice exhibited similar profiles to that observed in WT mice treated with BLM, with an increase in PA and a decrease in OA and linoleic acid (LA) compared with untreated WT. An elevation of PA and reduction of OA amount was exaggerated in Elovl6 −/− mice lung with BLM administration compared with WT mice, suggesting the role of Elovl6 as a key regulator of FA composition. Such a role of Elovl6 is most convincingly demonstrated in Elovl6 −/− mice treated with BLM. Several elongases and desaturases other than Elovl6 regulate FA composition. Thus, we measured mRNA expressions of Elovl5 , SCD1 , SCD2 , SCD3 and SCD4 in WT and Elovl6 −/− lungs, and found that BLM instillation significantly reduced Elovl5 gene expression in both WT and Elovl6 −/− lungs, whereas its expression was comparable between WT and Elovl6 −/− lungs at baseline ( Fig. 2g ). The alteration of the SCD gene expression in response to Elovl6 deletion or BLM instillation varied depending on SCD isoforms. The mRNA levels of SCD2 and SCD4 , but not SCD1 and SCD3 , were decreased in Elovl6 −/− lung at baseline, and BLM instillation significantly reduced the expression of the SCD2 , SCD3 and SCD4 . As shown in Fig. 2f , analyses of the lipid composition of the lung homogenate revealed that either Elovl6 deletion or BLM instillation decreased the proportion of C18:1n-9 (OA) as compared with that in WT lung homogenates. Although the relative contribution of SCD isoforms to desaturation process in mice lung remains to be explored, downregulation of Elovl5 , as well as of SCD2 and SCD4 , may at least partly explain the decrease in C18:1n-9 in Elovl6 −/− lung and BLM-instilled lung. Our data showed that LA content was significantly lower in Elovl6 −/− mice than in WT mice, although LA is not a major substrate for Elovl6. To address the mechanisms of a decrease of LA content in Elovl6 −/− lung, we measured mRNA levels of FA desaturase ( FADS ) 1 and 2 , which catalyse the desaturation reaction of n-6 polyunsaturated FA (PUFA), including LA [19] . Results showed that expression of the FADS1 and FADS2 genes was significantly reduced both in Elovl6 −/− and BLM-treated mice ( Fig. 2g ). Next, we examined mRNA expressions of FA transport proteins ( FATP ) 1 , 3 and 4 , which have a role in the uptake of long-chain FAs [20] , [21] . As shown in Fig. 2g , the expressions of the FATP1 , 3 and 4 genes were significantly reduced in mice treated with BLM, and FATP1 and 3 expressions were also significantly lower in Elovl6 −/− mice. Therefore, the decrease of LA content in Elovl6 −/− mice may be attributed to the impairment of the uptake of long-chain FAs through the downregulation of the FATP expressions. BLM induces apoptosis and TGF-β1 expression in the lung An important question is why Elovl6 −/− mice manifest pulmonary fibrosis at baseline and are highly susceptible to BLM compared with WT mice. One possible explanation is that Elovl6 deletion per se causes apoptosis of alveolar epithelial cells and/or induces TGF-β1 production in these cells, given that apoptosis and TGF-β1 production in alveolar epithelial cells largely contributes to the development of fibrosis [4] , [5] , [6] , [7] , [8] , [9] . Hence, we compared fluorescent TUNEL staining and caspase 3 activity between WT or Elovl6 −/− lungs before and after BLM instillation. As shown in Fig. 3a , representative immunofluorescence images showed that TUNEL-positive cells were detected in Elovl6 −/− mice but scarcely detected in WT mice before BLM instillation. Double immunofluorescent staining for TUNEL and SP-C together with DAPI (4',6-diamidino-2-phenylindole) staining of lung tissues from WT and Elovl6 −/− mice showed the colocalization of TUNEL-positive and SP-C-positive cells, indicating that TUNEL-positive cells are indeed alveolar type II epithelial cells ( Fig. 3b ). In addition, our data showed clearly that the number of TUNEL-positive cells was significantly increased in Elovl6 −/− mice compared with WT mice as early as 7 days and after BLM exposure ( Fig. 3c ). Moreover, western blot analysis of the lung homogenates revealed that cleaved-caspase 3 production levels were more increased in Elovl6 −/− mice compared with that in WT mice, and this effect was pronounced by the administration of BLM as early as 7 days ( Fig. 3d,e and Supplementary Fig. S1a ) and 21 days after BLM instillation ( Fig. 3f,g ). 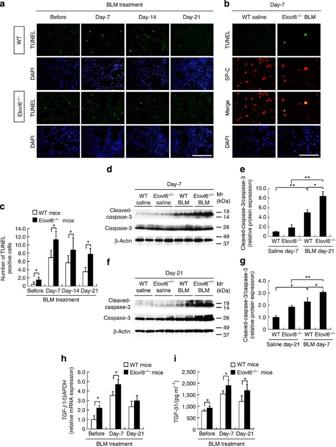Figure 3: Apoptosis and TGF-β1 expression are induced inElovl6−/−mouse lung exposed to BLM. (a) Representative immunofluorescence staining for TUNEL, and (c) the number of TUNEL-positive cells per high-power field in lung sections. TUNEL-positive cells were increased inElovl6−/−mice compared with WT mice, much further increased inElovl6−/−mice treated with BLM on days 7, 14 and 21, respectively. Scale bar, 200 μm.N=5–7 per group. Values are represented as the means±s.d. *P<0.05 versus WT before or BLM administration on each day, Student’st-test. (b) TUNEL labelling combined with anti-SP-C by immunohistochemistry.Elovl6−/−mice treated with BLM at 7 days showed that TUNEL-positive nuclei were colocalized with SP-C-positive cellular material in intra-alveolar cellular debris. Scale bar, 100 μm. (d–g) Western blotting analysis of cleaved-caspase 3 and total caspase 3 in the lung. Similar to TUNEL staining, cleaved-caspase 3 was increased inElovl6−/−mice compared with that in WT mice, further increased inElovl6−/−mice treated with BLM at 7 (d) and 21 days (f). Western blot data for cleaved-caspase 3 was normalized by total caspase 3 of the same sample and expressed fold increase compared with mean level of WT mice (e,g).N=4–6 per group. β-Actin was measured as an internal control. *P<0.05, **P<0.01 versus WT/Elovl6−/−treated with saline or BLM, Steel–Dwass test. (h) qRT–PCR forTGF-β1mRNA expression in the lungs. (i) The protein expression of TGF-β1 in lung tissues was measured by ELISA assay. The levels of TGF-β1 were significantly increased inElovl6−/−mouse lung before and after treatment with BLM compared with WT mouse lung on days 7 and 21, respectively.N=4–8 per group. Ine,g,handi, all values are represented as the means±s.d. of three experiments.GAPDHwas measured as an internal control. mRNA of the saline-treated group was normalized to a value of 1, and the mRNA levels in theElovl6−/−mice and BLM-treated group are shown relative to the control level. *P<0.05 versus WT before or BLM administration at that time point, Student’st-test. Figure 3: Apoptosis and TGF-β1 expression are induced in Elovl6 −/− mouse lung exposed to BLM. ( a ) Representative immunofluorescence staining for TUNEL, and ( c ) the number of TUNEL-positive cells per high-power field in lung sections. TUNEL-positive cells were increased in Elovl6 −/− mice compared with WT mice, much further increased in Elovl6 −/− mice treated with BLM on days 7, 14 and 21, respectively. Scale bar, 200 μm. N =5–7 per group. Values are represented as the means±s.d. * P <0.05 versus WT before or BLM administration on each day, Student’s t -test. ( b ) TUNEL labelling combined with anti-SP-C by immunohistochemistry. Elovl6 −/− mice treated with BLM at 7 days showed that TUNEL-positive nuclei were colocalized with SP-C-positive cellular material in intra-alveolar cellular debris. Scale bar, 100 μm. ( d – g ) Western blotting analysis of cleaved-caspase 3 and total caspase 3 in the lung. Similar to TUNEL staining, cleaved-caspase 3 was increased in Elovl6 −/− mice compared with that in WT mice, further increased in Elovl6 −/− mice treated with BLM at 7 ( d ) and 21 days ( f ). Western blot data for cleaved-caspase 3 was normalized by total caspase 3 of the same sample and expressed fold increase compared with mean level of WT mice ( e , g ). N =4–6 per group. β-Actin was measured as an internal control. * P <0.05, ** P <0.01 versus WT/ Elovl6 −/− treated with saline or BLM, Steel–Dwass test. ( h ) qRT–PCR for TGF-β1 mRNA expression in the lungs. ( i ) The protein expression of TGF-β1 in lung tissues was measured by ELISA assay. The levels of TGF-β1 were significantly increased in Elovl6 −/− mouse lung before and after treatment with BLM compared with WT mouse lung on days 7 and 21, respectively. N =4–8 per group. In e , g , h and i , all values are represented as the means±s.d. of three experiments. GAPDH was measured as an internal control. mRNA of the saline-treated group was normalized to a value of 1, and the mRNA levels in the Elovl6 −/− mice and BLM-treated group are shown relative to the control level. * P <0.05 versus WT before or BLM administration at that time point, Student’s t -test. Full size image We next performed qRT–PCR analysis of RNA from the lung and found that TGF-β1 mRNA levels were increased in Elovl6 −/− mice compared with WT mice at baseline, and was strongly augmented in BLM-treated Elovl6 −/− mice at day 7 and day 21 ( Fig. 3h ). In addition, the protein amount of TGF-β1 as assessed by enzyme-linked immunosorbent assay (ELISA; Fig. 3i ) was significantly increased in Elovl6 −/− lung before and after treatment with BLM compared with WT lung. These results were compatible with the results of TGF-β1 mRNA expression. Together, these results suggest that an induction of both apoptosis and TGF-β1 production in alveolar type II epithelial cells is an important mechanism for the exacerbation of BLM-induced pulmonary fibrosis in Elovl6 −/− mice. Elovl6 depletion alters FA composition in vitro To examine the effects of Elovl6 knockdown on FA composition in alveolar type II epithelial cells, we used a small interfering RNA (siRNA)-mediated approach to reduce Elovl6 gene expression in LA-4 cells, a cell line derived from murine alveolar type II epithelial cells. Elovl6 mRNA levels and elongase activity were significantly decreased in si Elovl6 -introduced LA-4 cells ( Fig. 4a,b ). Of note, Elovl6 depletion in LA-4 cells increased relative amounts of PA (C16:0) and decreased OA (C18:1n-9; Fig. 4c ). These changes were analogous to those observed in Elovl6 −/− mice. In addition, Elovl6 depletion in LA-4 cells significantly increased palmitoleic acid (C16:1n-7) and decreased stearic acid (C18:0), whereas LA (C18:2n-6) and arachidonic acid (C20:4n-6) were unchanged. Given that 18:2n-6 or 20:4n-6, long-chain FAs of the n-6 series, can only be synthesized from precursors from dietary precursors in vivo , the observation in Elovl6 -depleted LA-4 cells may not be relevant to the metabolism of 18:2n-6 or 20:4n-6 in Elovl6 −/− mice. However, these results indicate that Elovl6 depletion significantly changes FA composition in alveolar type II epithelial cells in a manner similar to that observed in Elovl6 −/− lung. 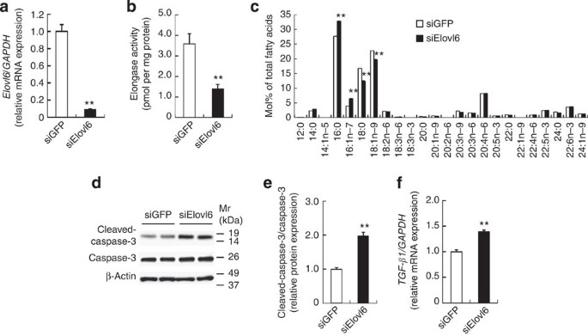Figure 4:Elovl6gene silencing in LA-4 cells induces apoptosis and TGF-β1 expression by alteration of FA composition. (a) qRT–PCR forElovl6gene expression and (b) Elovl6 enzymatic activity in LA-4 cells transfected withElovl6or green fluorescent protein (GFP) siRNA. TheElovl6siRNA robustly suppressedElovl6expression and activity compared with GFP siRNA. Specific activity was expressed as pmol of radioactive [2-14C] malonyl-CoA incorporated into hydrophobic long-chain FA fractions by 1 mg of microsomal protein.N=6 per group. (c) FA composition of neutral lipid extract from LA-4 cells. The transfection withElovl6siRNA increased relative amounts of PA (C16:0) and palmitoleic acid (C16:1n-7), decreased those of stearic acid (C18:0) and OA (C18:1n-9) compared with transfection with GFP siRNA (control) for 48 h.N=3 per group. (d,e) Western blotting analysis of cleaved-caspase 3 and total caspase 3 in LA-4 cells. Cleaved-caspase 3 was increased in siRNA-mediatedElovl6knockdown in comparison with siGFP transfection. Western blot data for cleaved-caspase 3 was normalized by total caspase 3 of the same sample, and expressed fold increase compared with mean level of siGFP group (e).N=6 per group. β-Actin was measured as an internal control. (f) qRT–PCR forTGF-β1mRNA expression in LA-4 cells.TGF-β1gene expression was significantly increased in siRNA-mediatedElovl6knockdown in comparison with siGFP transfection.GAPDHwas measured as an internal control. mRNA of the siGFP-treated group was normalized to a value of 1, and the mRNA levels inElovl6siRNA cells is shown relative to the control level.N=6 per group. In all data, values are represented as the means±s.d. of three experiments. **P<0.01 versus siGFP group, Mann–WhitneyU-test or Student’st-test (b). Figure 4: Elovl6 gene silencing in LA-4 cells induces apoptosis and TGF-β1 expression by alteration of FA composition. ( a ) qRT–PCR for Elovl6 gene expression and ( b ) Elovl6 enzymatic activity in LA-4 cells transfected with Elovl6 or green fluorescent protein (GFP) siRNA. The Elovl6 siRNA robustly suppressed Elovl6 expression and activity compared with GFP siRNA. Specific activity was expressed as pmol of radioactive [2- 14 C] malonyl-CoA incorporated into hydrophobic long-chain FA fractions by 1 mg of microsomal protein. N =6 per group. ( c ) FA composition of neutral lipid extract from LA-4 cells. The transfection with Elovl6 siRNA increased relative amounts of PA (C16:0) and palmitoleic acid (C16:1n-7), decreased those of stearic acid (C18:0) and OA (C18:1n-9) compared with transfection with GFP siRNA (control) for 48 h. N =3 per group. ( d , e ) Western blotting analysis of cleaved-caspase 3 and total caspase 3 in LA-4 cells. Cleaved-caspase 3 was increased in siRNA-mediated Elovl6 knockdown in comparison with siGFP transfection. Western blot data for cleaved-caspase 3 was normalized by total caspase 3 of the same sample, and expressed fold increase compared with mean level of siGFP group ( e ). N =6 per group. β-Actin was measured as an internal control. ( f ) qRT–PCR for TGF-β1 mRNA expression in LA-4 cells. TGF-β1 gene expression was significantly increased in siRNA-mediated Elovl6 knockdown in comparison with siGFP transfection. GAPDH was measured as an internal control. mRNA of the siGFP-treated group was normalized to a value of 1, and the mRNA levels in Elovl6 siRNA cells is shown relative to the control level. N =6 per group. In all data, values are represented as the means±s.d. of three experiments. ** P <0.01 versus siGFP group, Mann–Whitney U -test or Student’s t -test ( b ). Full size image Elovl6 depletion induces apoptosis and TGF-β1 expression We next tested whether Elovl6 deficiency by itself is causative for apoptosis and TGF-β1 expression in LA-4 cells. Results showed that Elovl6 knockdown induced caspase 3 activity ( Fig. 4d,e ) and TGF-β1 gene expression ( Fig. 4f ). These results indicate that Elovl6 deficiency is responsible for apoptosis and TGF-β1 production in LA-4 cells. PA induces apoptosis and TGF-β1 expression We examined the effects of PA on apoptosis and TGF-β1 production in LA-4 cells. PA induced caspase 3 activity ( Fig. 5a,b and Supplementary Fig. S1b ) and TGF-β1 mRNA expression ( Fig. 5c ) in a dose-dependent manner. Next, we performed costimulation with PA and OA, or LA in LA-4 cells. We found that OA and LA attenuated PA-induced apoptosis and TGF-β1 mRNA expression ( Fig. 5c–e ). These results are consistent with the hypothesis that alteration of FA composition, an increase in PA and a decrease in OA drives the induction of apoptosis and TGF-β1 in alveolar type II epithelial cells. 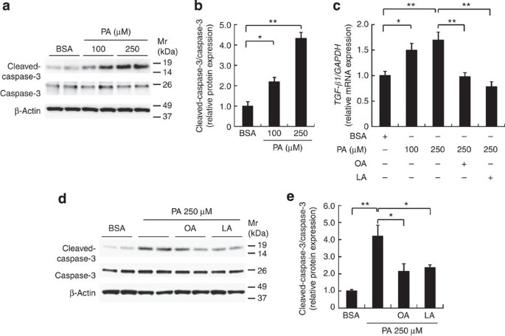Figure 5: OA and LA attenuate PA-induced apoptosis and TGF-β1 expression. (a,b) Western blotting analysis of cleaved-caspase 3 and total caspase 3 in LA-4 cells. Cleaved-caspase 3 was significantly increased in treatment (24 h) of PA (100–250 μM) in a dose-dependent manner. (c) qRT–PCR forTGF-β1mRNA expression in LA-4 cells. PA (100–250 μM) inducedTGF-β1gene expression in a dose-dependent manner, and costimulation of OA (250 μM) or LA (250 μM) significantly reduced PA-inducedTGF-β1mRNA expression.GAPDHwas measured as an internal control. mRNA of the BSA group was normalized to a value of 1, and the mRNA levels in cells treated with FA are shown relative to the control level.N=6–9 per group. (d,e) Costimulation of OA (250 μM) or LA (250 μM) significantly reduced PA-induced cleaved-caspase 3 expression in LA-4 cells. Western blot data for cleaved-caspase 3 was normalized by total caspase 3 of the same sample, and expressed fold increase compared with mean level of BSA group (b,e).N=6–8 per group. β-Actin was measured as an internal control. Inb,cande, values are represented as the means±s.d. of three experiments. *P<0.05, **P<0.01 versus BSA or PA group, Steel–Dwass test. Figure 5: OA and LA attenuate PA-induced apoptosis and TGF-β1 expression. ( a , b ) Western blotting analysis of cleaved-caspase 3 and total caspase 3 in LA-4 cells. Cleaved-caspase 3 was significantly increased in treatment (24 h) of PA (100–250 μM) in a dose-dependent manner. ( c ) qRT–PCR for TGF-β1 mRNA expression in LA-4 cells. PA (100–250 μM) induced TGF-β1 gene expression in a dose-dependent manner, and costimulation of OA (250 μM) or LA (250 μM) significantly reduced PA-induced TGF-β1 mRNA expression. GAPDH was measured as an internal control. mRNA of the BSA group was normalized to a value of 1, and the mRNA levels in cells treated with FA are shown relative to the control level. N =6–9 per group. ( d , e ) Costimulation of OA (250 μM) or LA (250 μM) significantly reduced PA-induced cleaved-caspase 3 expression in LA-4 cells. Western blot data for cleaved-caspase 3 was normalized by total caspase 3 of the same sample, and expressed fold increase compared with mean level of BSA group ( b , e ). N =6–8 per group. β-Actin was measured as an internal control. In b , c and e , values are represented as the means±s.d. of three experiments. * P <0.05, ** P <0.01 versus BSA or PA group, Steel–Dwass test. Full size image Elovl6 depletion and PA increase ROS generation To test whether an induction apoptosis and TGF-β1 expression by Elovl6 deficiency is mediated by ROS generation, we performed immunohistochemical staining for nitrotyrosine, a marker of oxidative stress [22] . Nitrotyrosine immunoreactivity was observed in alveolar epithelial cells in Elovl6 −/− mice but barely detected in WT mice before BLM instillation ( Fig. 6a ). Furthermore, nitrotyrosine-positive cells were increased in WT and Elovl6 −/− mice after BLM instillation ( Fig. 6a ). These findings suggest that lack of Elovl6 per se might result in increased ROS production in pulmonary alveolar epithelial cells. To test this hypothesis, we isolated primary alveolar type II epithelial cells from WT and Elovl6 −/− mice. Purity of alveolar type II epithelial cells was confirmed by immunofluorescence staining with anti-SP-C antibody ( Fig. 6b ) and Nile red staining ( Fig. 6c ). Next, we examined ROS production using CM-H 2 DCFDA (5-(6)-chloromethyl-2′,7′-dichlorodihydrofluorescein diacetate, acetyl ester) probe in these cells, and found that ROS production was detectable in alveolar type II epithelial cells from Elovl6 −/− mice but not from WT mice ( Fig. 6d ). In accordance with these results, Elovl6 knockdown induced ROS generation more prominently compared with LA-4 cells treated with green fluorescent protein controls ( Fig. 6e ). In addition, PA induced ROS generation and OA or LA inhibited PA-induced ROS production in LA-4 cells ( Fig. 6f ). 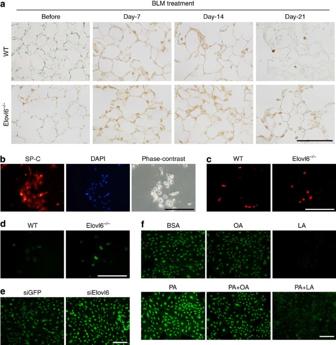Figure 6: ROS generation is increased inElovl6−/−mice or LA-4 cells treated withElovl6siRNA or PA. (a) Immunohistochemical staining with antibody against nitrotyrosine in lung sections. Positive staining cells were increased inElovl6−/−mouse compared with WT mouse, and the treatment of BLM also increased positive staining cells in WT mouse in comparison with that of saline. Furthermore, the number of positive staining cells was more increased inElovl6−/−mouse treated with BLM. Scale bar, 100 μm. (b,c) Alveolar type II epithelial cells were isolated from WT andElovl6−/−mice and maintained in culture for 48 h. (b) Immunofluorescence and phase-contrast images after staining with antibodies against SP-C in alveolar type II epithelial cell isolated fromElovl6−/−mouse. Expression of SP-C was localized with DAPI (4',6-diamidino-2-phenylindole) in alveolar type II epithelial cell. (c) Nile red staining showed that the dye was localized within the lamellar bodies in alveolar type II epithelial cells. (d–f) Intracellular ROS productions were detected using the oxidant-sensitive fluorogenic probe CM-H2DCFDA in primary alveolar type II epithelial cells from WT andElovl6−/−mice or LA-4 cells. (d) Alveolar type II epithelial cells fromElovl6−/−mice showed greater ROS fluorescence compared with level WT mice, and (e) siRNA-mediatedElovl6knockdown increased ROS level compared with siGFP transfection. (f) Stimulation with PA (250 μM) also increased ROS level in comparison with BSA, and costimulation of OA (250 μM) or LA (250 μM) reduced PA-induced ROS generation. Scale bar, 200 μm (b–f). Figure 6: ROS generation is increased in Elovl6 −/− mice or LA-4 cells treated with Elovl6 siRNA or PA. ( a ) Immunohistochemical staining with antibody against nitrotyrosine in lung sections. Positive staining cells were increased in Elovl6 −/− mouse compared with WT mouse, and the treatment of BLM also increased positive staining cells in WT mouse in comparison with that of saline. Furthermore, the number of positive staining cells was more increased in Elovl6 −/− mouse treated with BLM. Scale bar, 100 μm. ( b , c ) Alveolar type II epithelial cells were isolated from WT and Elovl6 −/− mice and maintained in culture for 48 h. ( b ) Immunofluorescence and phase-contrast images after staining with antibodies against SP-C in alveolar type II epithelial cell isolated from Elovl6 −/− mouse. Expression of SP-C was localized with DAPI (4',6-diamidino-2-phenylindole) in alveolar type II epithelial cell. ( c ) Nile red staining showed that the dye was localized within the lamellar bodies in alveolar type II epithelial cells. ( d – f ) Intracellular ROS productions were detected using the oxidant-sensitive fluorogenic probe CM-H 2 DCFDA in primary alveolar type II epithelial cells from WT and Elovl6 −/− mice or LA-4 cells. ( d ) Alveolar type II epithelial cells from Elovl6 −/− mice showed greater ROS fluorescence compared with level WT mice, and ( e ) siRNA-mediated Elovl6 knockdown increased ROS level compared with siGFP transfection. ( f ) Stimulation with PA (250 μM) also increased ROS level in comparison with BSA, and costimulation of OA (250 μM) or LA (250 μM) reduced PA-induced ROS generation. Scale bar, 200 μm ( b – f ). Full size image Oxidative stress downregulates Elovl6 expression BLM produces ROS in human lung [23] . Accordingly, we stimulated LA-4 cells with hydrogen peroxide (H 2 O 2 : 10 μM). H 2 O 2 treatment resulted in ~75% decrease in Elovl6 mRNA levels as assessed by qRT–PCR (relative mRNA expression of Elovl6 / GAPDH ; control 1.0±0.06 versus H 2 O 2 0.25±0.06, means±s.d., N =6 per group, P <0.01, Mann–Whitney U -test), suggesting that the Elovl6 gene expression is sensitive to ROS. Despite the considerable evidence that alveolar type II epithelial cells have a central role in phospholipid containing surfactant production, little attention has been paid for the regulation of lipid metabolism in these cells. In the present study, we provide several lines of evidence, indicating that the lack of Elovl6 has a causative role in lung fibrosis. First, apoptosis and ROS production were increased in Elovl6 −/− lung. Second, alveolar type II epithelial cells isolated from Elovl6 −/− mice and LA-4 cells produced increased levels of ROS. Third, Elovl6 deficiency increased PA and decreased OA and PUFA LA content in alveolar type II epithelial cells both in vivo and in vitro . Lastly, expressions of the genes for FADS1 , FADS2 , FATP s and FAT/CD36 were significantly reduced in Elovl6 −/− mice, suggesting that cellular uptake of long-chain FAs, including PUFA, was impaired in Elovl6 −/− mice. To our knowledge, this series of evidence allows us to propose that an alteration of lipid composition in alveolar type II epithelial cells in general and Elovl6 deficiency in particular impinge on the survival and function of alveolar type II epithelial cells, which have a crucial role in the maintenance of lung homeostasis. In addition, we show that Elovl6-mediated FA metabolism in the alveolar type II epithelial cells is perturbed in BLM-induced pulmonary fibrosis model, which could have important consequences in pulmonary pathology. We identified distinct expression of Elovl6 in alveolar type II epithelial cells in the normal adult mice lung, where it has the potential to regulate lipogenesis. Indeed, we found that Elovl6 −/− mice lung exhibited an increase in C16 PA and a decrease in C18 OA content. Furthermore, LA-4 cells treated with si Elovl6 showed an increase in both C16 PA and palmitoleic acid, and a decrease in both C18 stearic acid and OA. These findings were consistent with previous reports describing the effects of Elovl6 deficiency on hepatocytes and pancreatic β-cells [15] , [16] , [24] . Of particular interest, we note that C18:2n-6 (LA), an essential PUFA that can only be synthesized from dietary precursors, was decreased in Elovl6 −/− lung compared with those in WT lung. To understand the mechanisms underlying this observation, we examined the expression of the Elovl5 , FADS1 and FADS2 genes that promote the conversion of C18:2n-6 (LA) to C20:4n-6 (arachidonic acid). Results showed that FADS1 and FADS2 mRNA levels were significantly reduced in Elovl6 −/− lung and in BLM-treated mice lung. These results were contrary to our expectation, because a decrease in FADS1 and FADS2 expression is likely to cause an increase in C18:2n-6 (LA). Next, we examined the expression of the genes for FATPs and FAT/CD36 , all of which have a major role in the cellular uptake of long-chain FAs. As shown in Fig. 2g , the expression of the genes for FATP1 , 3 and 4 , and FAT/CD36 , was significantly, or tended to be, decreased in Elovl6 −/− mice and in BLM-treated mice lung. Although the molecular mechanisms underlying the decrease in the FATP1 , 3 and 4 , and FAT/CD36 , gene expression in Elovl6 −/− or BLM-treated mice lungs remain to be determined, these data suggest that a decrease in C18:2n-6 (LA) in Elovl6 −/− lung is largely due to a decrease in the uptake of long-chain FAs rather than the alteration of elongation and desaturation processes. From these in vivo and in vitro studies, an increase in C16 PA and/or a decrease in C18 OA in alveolar type II epithelial cells contribute to the pulmonary fibrosis in Elovl6 −/− mice. We demonstrated that Elovl6 deficiency resulted in exacerbation of pulmonary fibrosis in mice when they are exposed to BLM. A number of evidence established that BLM induced apoptosis in the alveolar epithelial and endothelial cells [25] , [26] , [27] , which has a key role in the initiation and progression of pulmonary fibrosis [28] . Indeed, we found the induction of apoptosis and caspase 3 activation in the lung from Elovl6 −/− mice, and confirmed them in Elovl6 -kockdown LA-4 cells. Therefore, it is likely to be that Elovl6 exerts its anti-apoptotic effect in alveolar type II epithelial cells. Our findings that PA induced caspase 3 activity in LA-4 cells, and either OA or LA attenuated PA-induced caspase 3 activity, are consistent with the previous reports described in a variety of cell types [29] , [30] , [31] , [32] , [33] , [34] , [35] . Therefore, we hypothesize that the increased apoptosis of alveolar type II epithelial cells in Elovl6 −/− mice is attributable to an increase in C16 PA and/or a decrease in C18 OA and C18 LA within the cells. A working hypothesis illustrated in Fig. 7 emphasizes the role of Elovl6 as a key regulator of the BLM-induced pulmonary fibrosis based on the findings of the present study and pertinent evidence from the previous studies. We found that Elovl6 deletion and BLM instillation induced prominent changes in gene expression involved in the synthesis and uptake of monounsaturated FA and PUFA. We showed that the expressions of the FATP1 , 3 and 4 , and FAT/CD36 , genes were significantly reduced in mice treated with BLM, and FATP1 and 3 expressions were decreased in Elovl6 −/− mice. Given that FATP1 , 3 and 4 , and FAT/CD36 , have an important role in the uptake of long-chain FAs from circulation, a decrease in the expression of these genes are likely to account for the decrease in the content of LA, a potent anti-apoptotic and anti-inflammatory lipid species, in Elovl6 −/− lung and BLM-treated lung. 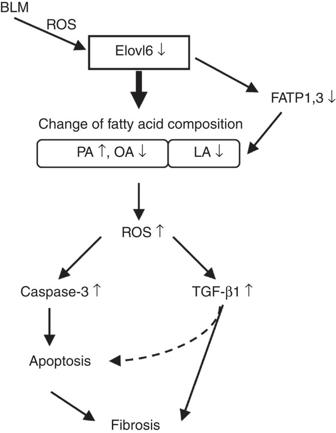Figure 7: Schematic diagram of pulmonary fibrosis caused byElovl6deficiency. BLM induces ROS generation in the lung, and oxidative stress downregulatesElovl6expression in alveolar epithelial cells. Subsequently, the loss of Elovl6 function induces the change of FA composition in which cytotoxic PA is increased and cytoprotective OA and LA are decreased in alveolar type II epithelial cells, resulting in increment of ROS generation, followed by induction of apoptosis and TGF-β1 expression. TheseElovl6deficiency induced inductions of ROS, apoptosis and TGF-β1 can progress BLM-induced pulmonary fibrosis. Figure 7: Schematic diagram of pulmonary fibrosis caused by Elovl6 deficiency. BLM induces ROS generation in the lung, and oxidative stress downregulates Elovl6 expression in alveolar epithelial cells. Subsequently, the loss of Elovl6 function induces the change of FA composition in which cytotoxic PA is increased and cytoprotective OA and LA are decreased in alveolar type II epithelial cells, resulting in increment of ROS generation, followed by induction of apoptosis and TGF-β1 expression. These Elovl6 deficiency induced inductions of ROS, apoptosis and TGF-β1 can progress BLM-induced pulmonary fibrosis. Full size image In addition, in concert with the abundant evidence indicating that ROS is central to BLM-induced pulmonary fibrosis [25] , [36] , [37] , [38] , our study demonstrate that alveolar type II epithelial cells in Elovl6 −/− mice produce more ROS than those in WT mice as assessed by staining with antibody against nitrotyrosine. These results help explain why Elovl6 −/− mice are more susceptible to BLM-induced pulmonary fibrosis. As excessive amount of extracellular matrix was synthesized and deposited in the lung of Elovl6 −/− mice treated with BLM, and as TGF-β1 has an indispensable role in the activation of alveolar epithelial cells and myofibroblasts, the key effector cells in fibrinogenesis [39] , [40] , we sought evidence for whether Elovl6 deficiency may induce TGF-β1 expression in alveolar cells. As expected, we found that TGF-β1 mRNA levels were increased in the lung of Elovl6 −/− mice in comparison with WT mice, and TGF-β1 gene expression was upregulated by siRNA for Elovl6 in LA-4 cell. Figure 7 illustrates these results. The potential mechanisms underlying the upregulation of TGF-β1 expression in Elovl6 -deficient cells also warrant consideration. We found that exposure of LA-4 cells to PA induced TGF-β1 mRNA expression in a dose-dependent manner, and this response was blunted in the presence of OA and LA in the culture medium. These observations were consistent with the previous reports using pancreatic β-cell line [41] . Toll-like receptor 4-dependent and -independent signalling pathways have been documented to mediate the response to extracellular FAs. In addition, there has been much evidence indicating that intracellular FAs regulate the gene expression, at least partly through the generation of ROS and ligands for peroxisome proliferator-activated receptor or liver X receptor family receptors, as do the exogenously supplied FAs exert their effects after they are taken up in the cells [42] , [43] , [44] . Thus, it seems reasonable to speculate that an increase in PA relative to OA and LA levels within the alveolar type II epithelial cells is responsible for the induction of TGF-β1. Further studies are required to determine to what extent signalling pathways leading to TGF-β1 gene induction overlap between the stimuli with exogenous and endogenous FAs. Our findings that dysregulation of lipid metabolism in alveolar type II epithelial cells due to Elovl6 deficiency contributes to pulmonary fibrosis has an important clinical relevance. Diabetes has been described as a risk factors associated with pulmonary fibrosis. Usuki et al . [45] revealed that hyperglycaemia influenced the severity of pulmonary fibrosis in diabetic mice treated with BLM. In addition, Miyake et al . [46] demonstrated that intake of saturated FA and meat was associated with a 6.3- and 7.2-fold increased risk of IPF, respectively. Given that Elovl6 gene expression is downregulated upon exposure to hydrogen peroxide, we assume that predisposition to pulmonary fibrosis of the patients with diabetes or overnutrition may be attributed to the susceptibility of Elovl6 expression to oxidative stress. Indeed, immunohistochemistry of human lung tissue revealed that Elovl6 expression was barely detectable in IPF patients. In conclusion, this study allow us to propose novel mechanisms of pulmonary fibrosis by which derangement of Elovl6-mediating FA balance initiates ROS production and apoptosis in alveolar type II epithelial cells, and have an important role in BLM-induced pulmonary fibrosis. These findings reveal a previously unappreciated role of lipid composition in alveolar type II epithelial cells in the pulmonary pathophysiology. Future research will need to establish whether Elovl6 may be a potential target for the treatment of IPF. Reagents Kaighn’s F-12K Nutrient Mixture was purchased from Invitrogen (Carlsbad, CA). Fetal bovine serum was from Biowest (Nuaille, France). Elovl6 antibody was purchased from ABGENT (San Diego, CA), SP-C antibody was from Santa Cruz Biotechnology (Santa Cruz, CA); cleaved-caspase 3, caspase 3, nitrotyrosine and β-actin were from Cell Signaling Technology (Beverly, MA). FA-free BSA, PA and BSA-conjugated OA and LA solution were purchased from Sigma-Aldrich. Hydrogen peroxide (50 μM) was from Wako (Osaka, Japan). Mice Elovl6 −/− mice were a kind gift from Dr H. Shimano (Tsukuba University). These mice were intercrossed with Elovl6 −/− or Elovl6 −/+ mice. Littermates were genotyped by PCR. Eight-week-old male WT and Elovl6 −/− mice were anaesthetized and instilled with BLM (1 mg kg −1 ) intratracheally using a microsprayer (Penn-Century, Philadelphia, PA) as described previously [47] . Control mice received saline. Mice were killed at 7, 14 and 21 days after BLM administration. Tissue preparation Following the incubation of deep anaesthesia, mice were killed and the left lungs were ligated and excised immediately. Tissue was frozen rapidly and stored at −70 °C until qRT–PCR and western blot analysis. The right lungs were inflated by instilling with 10% formalin at a constant pressure of 25-cm formalin for 10 min and fixed for 24 h before paraffin embedding. Human lung tissues were obtained from patients at autopsy and tissue samples were fixed in formalin and embedded in paraffin. Each serial section (4 μm) was prepared for histological analysis. Immunohistochemistry Sections were deparaffinized in xylene and rehydrated before antigen retrieval by boiling in citrate buffer. Elovl6, SP-C and nitrotyrosine stainings were performed using the Vectastatin Elite ABC kit (Vector Laboratories, Burlingame, CA) according to the manufacture’s instruction, with 3,3′-diaminobenzidine as the chromogenic substrate. Sections were stained with haematoxylin and eosin or Masson’s trichrome using standard procedures. Masson’s trichrome staining was used to detect fibrosis in lung sections, and the percentage of fibrosis areas were calculated as previously described [48] using ImageJ software (National Institutes of Health). Briefly, the histological sections were captured using an Olympus IX70 inverted microscope (Olympus, Tokyo, Japan). The images coloured by Masson’s trichrome blue were extracted and quantified in percentage in the area of each samples. The grade of pulmonary fibrosis in the lung sections was scored on a scale of 0–8 using Ashcroft scoring method [49] . The severity of fibrotic changes in each histological section of the lung was assessed as the mean score of severity from observed microscopic fields. After the examination of 30 randomly chosen regions in each sample at a magnification of × 100, the mean score of all the fields was taken as the fibrosis score. Grading was done in a blinded manner by three observers. RNA isolation and qRT–PCR Total RNA was extracted from the mouse lung tissue and LA-4 cell using ISOGEN regent (Takara Bio, Kyoto, Japan) according to the manufacturer’s protocol. One microgram of RNA was used for reverse transcription with the RNA LA PCR Kit (Takara Bio) and qRT–PCR analysis was performed using THUNDERBIRD SYBR qPCR Mix (TOYOBO, Osaka, Japan) according to the manufacturers’ protocol. qRT–PCR analysis was carried out using a MX3000P quantitative system (Stratagene, La Jolla, CA). All primer sequences are shown in Supplementary Table S1 . Three samples were used, respectively, for each of the three experiments performed. Elongase activity Microsomal FA elongation activity was assayed by the measurement of [2- 14 C]-malonyl-CoA incorporation into exogenous acyl-CoAs as described previously [15] , with some modification. Briefly, the assay mixtures contained 100 μM Tris-HCl, pH 7.4, 60 μM palmitoyl-CoA, 500 μM NADPH and freshly obtained microsomal protein, all in a final volume of 0.25 ml. After 2 min of preincubation at 37 °C, the reaction was started by the addition of 60 μM malonyl-CoA (containing 0.037 μCi of [2- 14 C] malonyl-CoA). After 10 min incubation at 37 °C, the reaction was stopped by addition of 0.5 ml of 10% KOH in methanol and saponified at 65 °C for 1 h. After acidification with 0.5 ml of ice-cold 5 N HCl, the free FAs were extracted from the mixture three times with 1 ml of hexane (total volume, 3 ml). The pooled hexane fractions were dried, and after addition of 3 ml of scintillation mixture the radioactivity incorporated was counted in a scintillator counter (Aloca LSC3000). Blanks were measured in parallel reactions incubated without microsomal fractions. Collagen assay The Sircol assay (Biocolor Ltd, Belfast, UK) was carried out following the manufacturer’s instructions. Briefly, the lung tissue was homogenized and total collagen was solubilized in 0.5 M acetic acid. Next, sirius red reagent was added to each lung homogenate and mixed for 30 min. The collagen–dye complex was precipitated by centrifugation at 12,000 r.p.m. for 10 min and dissolved in 0.5 M NaOH. Finally, the sample’s absorbance was determined at 540 nm and compared with a calibration curve generated using the collagen standard provided by the manufacturer. FA composition Lipids from mouse whole lung and LA-4 cell were extracted by Bligh and Dyer method [50] . Briefly, lung tissues and cells were extracted with chloroform/methanol (1:2, v/v) solution. One molar NaCl solution and chloroform were added to break the monophase and incubated on ice for 10 min. After centrifugation at 2,000 r.p.m. for 5 min, aqueous solution was discarded and chloroform phase was transferred to test tube. Chloroform phase was evaporated using nitrogen gas and the obtained lipids were requested for FA composition analysis to an external laboratory (SRL Inc., Tokyo, Japan). TUNEL staining For labelling nuclei of apoptotic cells, sections were stained with TUNEL method using the In Situ Cell Death Detection Kit, Fluorescein (Roche, Indianapolis, IN) according to the manufacturer’s protocol. Western blot analysis Tissue samples and cells were homogenized on ice in RIPA buffer (20 mM Tris-HCl (pH 7.4), 150 mM NaCl, 1% NP-40, 1% sodium deoxycholate and 0.1% SDS, and containing complete mini and phosSTOP solution (Roche). The mixture was centrifuged at 15,000 r.p.m. for 30 min and supernatant was subjected to SDS–PAGE. Protein concentrations were determined by the Bradford method using a colorimetric assay (Bio-Rad, Hercules, CA). Western blot analysis was performed according to standard procedures using the following primary antibodies: rabbit monoclonal cleaved-caspase 3 (Cell Signaling Technology, catalogue number 9664, 1:250), caspase 3 (Cell Signaling Technology, catalogue number 9665, 1:250) and β-actin (Cell Signaling Technology, catalogue number 4970, 1:500). Antigens were revealed by Immobilon Western HRP Substrate (Millipore, Billerica, MA) after incubation with horseradish peroxidase-conjugated anti-rabbit IgG. The band’s density was quantified using ImageJ software. ELISA assay for TGF-β1 The protein level of TGF-β1 in the mouse lung tissue was measured using an ELISA kit (R&D Systems, Minneapolis, MN). The protocol followed the manufacturer’s instructions. Total TGF-β1 levels were determined by acid activation (1 M hydrochloric acid, 10 min, room temperature) of the latent TGF-β1 in the homogenate. Preparation of FA solution PA was conjugated to FA-free BSA at a 3.5:1 molar ratio by dissolving them in ethanol and mixing with an aqueous BSA solution (BSA in PBS) at 37 °C until homogeneous, after which they were passed through a 0.2-μM filter. Culture of LA-4 cells Mouse lung type II epithelial cells (LA-4) were obtained from ATCC. LA-4 cells were cultured using Kaighn’s F-12 K Nutrient Mixture supplemented with 10% fetal bovine serum and 1% penicillin/streptomycin in a 5% CO 2 atmosphere at 37 °C. Serum-starved LA-4 cells with 0.1% BSA (24 h) were incubated in the presence or absence of BSA-conjugated PA, OA and LA (100–250 μM each). To examine the regulation of Elovl6 mRNA expression, hydrogen peroxide (50 μM) was also stimulated. After 24 h incubation at 37 °C, mRNA or protein was collected from the cells. Isolation of alveolar type II epithelial cells Alveolar type II epithelial cells were isolated from Elovl6 −/− and WT C57BL/6 mice, as described [51] , with minor modifications [52] . Briefly, the lungs were perfused with PBS injected through the right ventricle until the lungs were cleared of blood. Two millilitres of dispase (50 U ml −1 ; BD Biosciences, San Jose, CA) were instilled into the lungs and the syringe was left in place to prevent leakage of dispase. The lungs were then removed and transferred in 1 ml dispase for 45 min at room temperature. Lung tissue was separated from large bronchi by mechanical means with forceps and transferred to 5 ml of DMEM with 0.01% DNase I (Sigma-Aldrich) in a 60-mm culture plate, and chopped into fine pieces, followed by 10-min incubation at 37 °C. This crude preparation was filtered through 100-, 40- and 20-μm cell strainers (Millipore), and centrifuged at 1,000 r.p.m. for 10 min at 4 °C. The cell pellet was resuspended in 10 ml of DMEM with 10% FBS and placed on anti-CD45- (BD Bioscience) and anti-CD32- (BD Bioscience) coated petri dishes at 37 °C for 1 h to remove adherent macrophages. The unbound cells were collected and inoculated into non-coated culture plates at 37 °C for 1 h to remove adherent fibroblast. The remaining cells were collected and centrifuged (1,000 r.p.m. for 10 min). The pellet was resuspended in tissue culture medium consisting of DMEM/F-12 (Life Technologies), 1 mM L -glutamine, 10 mM Hepes, 0.25% BSA (Sigma-Aldrich), 5% mouse serum (Equitech-Bio, Kerrville, TX), 0.1 mM non-essential amino acids (Life Technologies), 0.05% insulin–transferrin–sodium selenite (BD Bioscience) and 1% penicillin–streptomycin (Life Technologies). The cells were then seeded on type I collagen-coated eight-well slide glass and maintained at 37 °C with 10% CO 2 . After 24 h, cells were washed and medium was replaced with serum-free medium. The isolated alveolar type II epithelial cells were confirmed by immunofluorescence staining using anti-SP-C antibody purchased from Santa Cruz Biotechnology. Secondary staining was performed with Cy3-conjugated anti-rabbit IgG. Alveolar type II epithelial cells were also identified by staining with modified Nile red (Wako), a lipophilic fluorescent dye that can label cellular lipid droplet in alveolar type II epithelial cells isolated from WT and Elovl6 −/− mice. Nile red, dissolved in dimethylsulphoxide, was added to unfixed cells in PBS (5 μg ml −1 ) and incubated for 10 min at room temperature to label the cells. The cells were washed with PBS, fixed with 4% paraformaldehyde and examined using fluorescence microscope. For each experiment, alveolar type II epithelial cells were 95% pure as confirmed by immunofluorescence staining for SP-C and the presence of Nile red-positive vacuoles. Construction of siRNA oligonucleotide and transfection siRNA oligonucleotides (mouse siElovl6: 5′-CGU CAU GUA CUC UUA CUA CGC-3′, siGFP: 5′-GUU CAG CGU GUC CGG CGA GTT-3′) were purchased from BONAC Corporation (Fukuoka, Japan) and transfected with Lipofectamine RNAiMAX Regent (Invitrogen) according to the manufacturer’s protocol. Estimation of ROS generation Intracellular ROS levels were detected with the oxidant-sensitive fluorogenic probes CM-H 2 DCFDA (Invitrogen Life Technologies). Isolated alveolar type II epithelial cells from Elovl6 −/− and WT mice were incubated with 1 μM CM-H 2 DCFDA in serum-free medium for 5 min at 37 °C. siRNA-transfected LA-4 cells were incubated with 10 μM CM-H 2 DCFDA in serum-free medium for 30 min at 37 °C. Next, the cells were incubated in the presence or absence of PA, OA and LA for 15 min. After incubation at 37 °C, fluorescence was detected. Statistical analysis All data are shown as mean±s.d. Two-group comparison was analysed by Mann–Whitney U -test or unpaired Student’s t- test, and multiple-group comparison was performed by one-way analysis of variance with Steel–Dwass or Tukey–Kramer’s multiple comparison tests. A P -value <0.05 was considered significant. Ethical approval Animal experiments using these mice were approved by and performed according to the guidelines of the Committee of Experimental Animal Research of Gunma University (permit number: 10-019). Human lung tissues were obtained from patients at autopsy with written informed consent of their family at the Gunma University Hospital. This protocol was approved by the Institutional Review Board at the Gunma University Hospital. How to cite this article: Sunaga, H. et al . Deranged fatty acid composition causes pulmonary fibrosis in Elovl6 -deficient mice. Nat. Commun. 4:2563 doi: 10.1038/ncomms3563 (2013).